Magneto-orbital helices as a route to coupling magnetism and ferroelectricity in multiferroic CaMn7O12 Orbital physics drives a rich phenomenology in transition-metal oxides, providing the microscopic underpinning for effects such as Colossal Magnetoresistance. In particular, magnetic and lattice degrees of freedom are coupled through orbital ordering, and it has long been hoped that this coupling could be exploited to create high-temperature multiferroics with large values of the electrical polarization. Here we report an unprecedented magneto-orbital texture in multiferroic CaMn 7 O 12 , found to give rise to the largest magnetically induced ferroelectric polarization measured to date. X-ray diffraction characterization of the structural modulation in these ‘magneto-orbital helices’, and analysis of magnetic exchange shows that orbital order is crucial in stabilising a chiral magnetic structure, thus allowing for electric polarization. Additionally, the presence of a global structural rotation enables the coupling between this polarization and magnetic helicity required for multiferroicity. These novel principles open up the possibility of discovering new multiferroics with even larger polarization and higher transition temperatures. Orbital ordering (OO) is one of the most striking manifestations of electronic correlations in a variety of materials, most notably in 3d transition-metal oxides [1] . In these systems, below a certain temperature T OO , a distinct anisotropic pattern of orbital occupation emerges from a nearly isotropic high-temperature state. As OO is strongly connected with both structural distortions (the cooperative Jahn Teller effect) and with magnetism, OO has long been regarded as a promising ingredient to allow the cross-coupling of electric properties. Recently, it has been proposed that some charge and orbitally ordered states could be electrically polar, so that OO could promote high-temperature, magnetically controllable ferroelectricity [2] . Here we show that a unique form of incommensurate OO in the complex manganese oxide CaMn 7 O 12 , appearing below 250 K, is responsible for the largest observed magnetically induced ferroelectric polarization. Unlike all other known systems, orbital occupation in CaMn 7 O 12 does not select fixed preferential directions, but rotates around the threefold crystallographic axis, preserving the overall point-group symmetry. The resulting pattern of magnetic exchange interactions produces a magnetic helix having twice the period of the orbital modulation below 90 K. Upon cooling below ∼ 400 K, CaMn 7 O 12 adopts a trigonal structure (space group ), shown in Fig. 1a . It can be described as a perovskite superstructure, with 3/4 of the A sites occupied by Mn 3+ (hereafter labelled Mn1), and the remaining occupied by Ca. The pseudocubic B sites form three inequivalent triangular layers stacked along the hexagonal c axis (shown in Fig. 1a , and coloured green, blue and red throughout this report). Within each layer, 1/4 of the B sites retain symmetry (Mn3, black-outlined circles in Fig. 1a ), whereas the other 3/4 have symmetry (Mn2). Charge ordering develops gradually on further cooling, with Mn2 and Mn3 tending towards Mn 3+ and Mn 4+ , respectively. An incommensurate structural modulation along the hexagonal c axis appears below T OO =250 K, with a propagation vector q c =(0, 0, 2.077±0.001) at 150 K, producing a continuous variation in Mn-O bond lengths [3] . 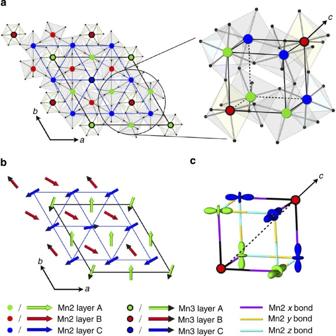Figure 1: The crystal and magnetic structures and associated orbital orientations of CaMn7O12. (a) (left panel) The room temperature crystal structure in the hexagonal setting, highlighting the three triangular layers (A, blue, B, red and C, green) stacked along the hexagonalcaxis (cubic [111] direction). The structure can also be described within the pseudocubic perovskite setting (right panel), with Mn3 sites (black-outlines spheres, with nominal valence 4+) occupying the apex sites along the [111] diagonal. (b) The magnetic structure at 90 K. The triangular layers are again shown as blue, red and green, with a 124° spin rotation between adjacent layers. (c) A schematic showing the B sites in the pseudocubic setting, defining thex,yandzbond directions, which are used to describe orbital orientation. Figure 1: The crystal and magnetic structures and associated orbital orientations of CaMn 7 O 12 . ( a ) (left panel) The room temperature crystal structure in the hexagonal setting, highlighting the three triangular layers (A, blue, B, red and C, green) stacked along the hexagonal c axis (cubic [111] direction). The structure can also be described within the pseudocubic perovskite setting (right panel), with Mn3 sites (black-outlines spheres, with nominal valence 4+) occupying the apex sites along the [111] diagonal. ( b ) The magnetic structure at 90 K. The triangular layers are again shown as blue, red and green, with a 124° spin rotation between adjacent layers. ( c ) A schematic showing the B sites in the pseudocubic setting, defining the x , y and z bond directions, which are used to describe orbital orientation. Full size image The magnetic structure below T N1 =90 K was determined using neutron powder diffraction [4] , and is shown in Fig. 1b . Magnetic anisotropy results in the spins lying within the hexagonal ab plane. Within each of the triangular layers, Mn2 spins are parallel to each other, while Mn3 spins are approximately antiparallel. Adjacent layers are rotated by 124° in the ab plane with respect to each other, leading to an incommensurate magnetic modulation with propagation vector q m =(0, 0, 1.037). As observed in many magnetically ordered crystals (see, for example [5] ), below T N1 , q c =2 q m . Here the structural modulation is also present in the paramagnetic phase, and the magnetic modulation ‘locks in’ to it as it develops at T N1 . Below T N2 =50 K, another magnetic transition occurs, with the appearance of a second propagation vector [4] . Sławiński et al. [6] have shown that the average propagation vector is constant across T N2 , and described the low-temperature magnetic phase as a ‘beating’ of the high-temperature phase—a model that provides a good fit to their neutron data. Although the origin of such complex low-temperature structure remains obscure, its symmetry properties (in particular its chirality) are very similar to the high-temperature phase, and the transition at T N2 has clearly very little effect on the electrical properties [4] . In this paper, we discuss primarily the simpler magnetic phase between T N1 and T N2 . In this phase, the magnetic structure induced by the orbital texture breaks inversion symmetry and couples to the crystal structure via the relativistic antisymmetric exchange to yield the large switchable electrical polarization. The structural modulation We now focus on the incommensurate structural modulation appearing below T OO , and demonstrate that this corresponds to the onset of a novel form of OO. Single-crystal X-ray diffraction data were measured at 150 K. Many different crystals from different batches were tested, consistently yielding sharp superstructure peaks, indicative of a long-range-ordered modulated structure. The modulated structure was refined using JANA 2006 [7] . Consistent with previous reports [3] , we found that the modulated crystal structure is described by the centrosymmetric four-dimensional space group (00γ)0 with propagation vector q c =(0, 0, 2.077). In Fig. 2a , we plot the Mn-O bond lengths for adjacent unit cells along the c axis around Mn2 (for variation in the Mn1-O and Mn3-O bond lengths see Supplementary Fig. S1 ). This structural modulation has strong implications for the nature of orbital occupation as follows. We define orthogonal x , y and z bond directions, schematically shown in Fig. 1c . In the unmodulated, average structure, the Mn 3+ O 6 octahedra around Mn2 are compressed, giving two short and four long bonds, implying an unusual occupation of the x 2 − y 2 orbital. In reality, the structural modulation leads to an incommensurate rotation of a single pair of long bonds in the xy plane. We can characterize this orbital rotation by employing a formalism first proposed by Goodenough [8] , [9] , which quantifies orbital occupation according to a mixing angle, . Following the conventions in Wu et al. [9] , we need only to consider the angular sector 2 π /3≤ θ ≤4 π /3 (inset to Fig. 2 ). As shown in Fig. 2b , the orbital occupation rotates periodically between the 3 x 2 − r 2 and 3 y 2 − r 2 orbitals, passing through the x 2 − y 2 only at the nodal points. Fig. 2c shows the Mn2 charge modulation accompanying the orbital modulation, calculated using the Bond Valence Sum method [10] . Valence fluctuations are surprisingly small (1%—see Supplementary Fig. S2 and Supplementary Discussion ), and may even be entirely an artefact of the model that does not account for the modulation of thermal parameters. This indicates that the character of the modulation is predominantly orbital. 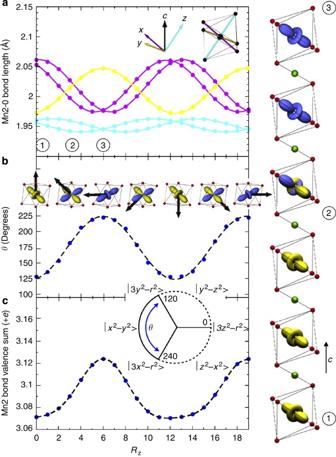Figure 2: The incommensurate structural modulation coupled to orbital rotation and valence fluctuations. (a) Variation in Mn2-O bond lengths alongx,yandz(coloured according to the schematic inFig. 1c) as a function ofRz, plotted across 19 unit cells along thecaxis. (b) Orbital mixing angleθfor the Mn2 octahedra as a function ofRz.θcorrelates directly with orbital occupation, as shown by the circular inset. The orbital rotation is shown, along with the coupled helical spin rotation. (c) The Mn2 charge modulation, which accompanies the structural modulation along thecaxis. The incommensurate orbital modulation for half a period of the structural modulation is depicted at the side of the figure, with positions 1, 2 and 3 corresponding to the labelled points in (a). Figure 2: The incommensurate structural modulation coupled to orbital rotation and valence fluctuations. ( a ) Variation in Mn2-O bond lengths along x , y and z (coloured according to the schematic in Fig. 1c ) as a function of R z , plotted across 19 unit cells along the c axis. ( b ) Orbital mixing angle θ for the Mn2 octahedra as a function of R z . θ correlates directly with orbital occupation, as shown by the circular inset. The orbital rotation is shown, along with the coupled helical spin rotation. ( c ) The Mn2 charge modulation, which accompanies the structural modulation along the c axis. The incommensurate orbital modulation for half a period of the structural modulation is depicted at the side of the figure, with positions 1, 2 and 3 corresponding to the labelled points in ( a ). Full size image The magneto-orbital helix Although OO is a widespread phenomenon [11] , [12] , an incommensurate modulation where the orbital occupation rotates perpendicular to the propagation direction is unprecedented. The resulting orbital arrangement has a profound effect on magnetic ordering below T N =90 K. This can be seen by applying the Goodenough–Kanamori–Anderson (GKA) rules [13] , [14] , [15] , [16] , which predict the nature of exchange interactions. In the absence of the structural modulation, the pseudo-perovskite structure is heavily distorted, and antiferromagnetic interactions are weak due to the large departure of the Mn-O-Mn bond angles from 180°. The alternation of filled and empty x 2 − y 2 orbitals on Mn2 and Mn3 promotes ferromagnetic exchange, and a net ferromagnetic structure is predicted. This is confirmed by first-principle calculations [17] , which also show that a rotating magnetic structure would require spin–orbit coupling. The situation changes drastically in the presence of the orbital modulation, which enables the helical magnetic structure to be stabilised by Heisenberg exchange and to lock to the superstructure. This is because the magnetic interaction between adjacent A, B and C layers is predominantly mediated by the orbitals that are most affected by the modulation, which introduces magnetic frustration. This is shown schematically in Fig. 3a , which depicts a region of the crystal structure where the modulation amplitude is largest. Mn3 in the B layer is connected to the Mn2 sites in the A layer by filled 3 x 2 − r 2 orbitals, yielding a ferromagnetic interaction J 1 , and to the Mn2 sites in the C layer by empty orbitals, yielding an antiferromagnetic interaction J 2 (crucially, J 1 and J 2 would be equal in the absence of OO). This produces an effective ferromagnetic interaction between spins in each of the A, B and C layers, as all J 1 ( J 2 )’s are equivalent by symmetry (shown in Fig. 3b ). Across layers there is an effective next-nearest-neighbour antiferromagnetic interaction J 12 , which is strongest at the ‘crest’ of the modulation, but remains antiferromagnetic everywhere except possibly at the nodal point. The overall nearest-neighbour interaction between layers, J 3 , results from the competition between full-empty ( x − z ) orbitals and empty-empty ( y − z ) orbitals, which are ferro- and antiferromagnetic, respectively. Although the sign of J 3 cannot be predicted a priori , it is experimentally found to be positive (antiferromagnetic). The magnetic helix, therefore, results from the competition between antiferromagnetic nearest-neighbour and next-nearest-neighbour interactions. We can test this hypothesis with a very simple model, which captures the effect of the average interactions J 1 , J 2 and J 3 , assuming a magnetic propagation vector (0,0, q z ) and identical spins S on Mn2 and Mn3 sites. 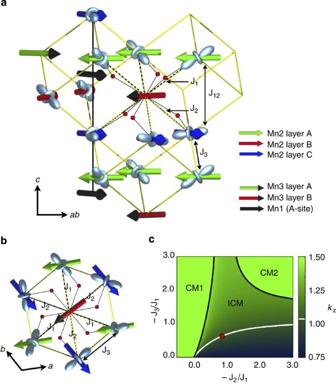Figure 3: The effect of OO on magnetic exchange interactions promotes a chiral magnetic structure. (a) Three pseudocubic unit cells illustrating the coupling between the incommensurate orbital modulation and the magnetic structure. The occupied Mn2 (Mn3+) orbitals are shown in grey, giving rise to ferromagnetic exchange interactions (J1), shown by a dashed line, and antiferromagnetic exchange interactions (J2), shown by a dotted line. The nearest-neighbour and effective next-nearest-neighbour antiferromagnetic exchanges between layers are labelledJ3andJ12, respectively. The ferromagnetic exchange along the Mn1–Mn2 chains is shown by a solid black line. (b)Figure 3aviewed down thecaxis, showing the symmetry equivalent exchange interactions. (c) Phase diagram of the CaMn7O12magnetic structures, obtained by minimizing the classical Heisenberg exchange energy in equation 1 as a function of the anglesψandφfor different exchange constantsJ1,J2andJ3. Spins on Mn2 and Mn3 sites were taken to be equal (different spins would be equivalent to renormalising the exchange constants). CM1 and CM2 are two commensurate collinear phases, both with propagation vector (0, 0, 1.5), in which the Mn2 and Mn3 in each layer are antiparallel (for CM1) and parallel (for CM2). ICM is an incommensurate phase with rotating spins (magnetic helix). The shading indicates the value of thez-component of the propagation vector. The white line indicates the locus of points with the experimental propagation vector (0, 0, 1.037). The red dot corresponds to the experimental magnetic structure (φ=31°). The magnetic Heisenberg exchange energy per Mn3 site can be written as: Figure 3: The effect of OO on magnetic exchange interactions promotes a chiral magnetic structure. ( a ) Three pseudocubic unit cells illustrating the coupling between the incommensurate orbital modulation and the magnetic structure. The occupied Mn2 (Mn 3+ ) orbitals are shown in grey, giving rise to ferromagnetic exchange interactions ( J 1 ), shown by a dashed line, and antiferromagnetic exchange interactions ( J 2 ), shown by a dotted line. The nearest-neighbour and effective next-nearest-neighbour antiferromagnetic exchanges between layers are labelled J 3 and J 12 , respectively. The ferromagnetic exchange along the Mn1–Mn2 chains is shown by a solid black line. ( b ) Figure 3a viewed down the c axis, showing the symmetry equivalent exchange interactions. ( c ) Phase diagram of the CaMn 7 O 12 magnetic structures, obtained by minimizing the classical Heisenberg exchange energy in equation 1 as a function of the angles ψ and φ for different exchange constants J 1 , J 2 and J 3 . Spins on Mn2 and Mn3 sites were taken to be equal (different spins would be equivalent to renormalising the exchange constants). CM1 and CM2 are two commensurate collinear phases, both with propagation vector (0, 0, 1.5), in which the Mn2 and Mn3 in each layer are antiparallel (for CM1) and parallel (for CM2). ICM is an incommensurate phase with rotating spins (magnetic helix). The shading indicates the value of the z -component of the propagation vector. The white line indicates the locus of points with the experimental propagation vector (0, 0, 1.037). The red dot corresponds to the experimental magnetic structure ( φ =31°). Full size image where ψ =2/3 πq z and φ are the angles between Mn2-Mn2 and Mn3-Mn2 spins in adjacent layers, respectively. Minimizing the energy in equation 1 yields the phase diagram shown in Fig. 3c . The wide incommensurate phase field is bound on either side by two distinct commensurate collinear phases, both with q z =1.5. The white line indicates the range of parameters for which the most stable propagation vector is that determined experimentally. The red dot corresponds precisely to the experimental magnetic structure ( φ =31°), and is found for J 2 / J 1 =−0.85 and J 3 / J 1 =−0.63, in good agreement with our qualitative considerations based on the GKA rules. The coupling between Mn1 and adjacent Mn2 sites is expected (and observed) to be ferromagnetic ( Fig. 3a ) as the sites are linked via oxygen anions with highly-distorted bonds at less than the GKA critical angle. The most important ingredient not included in our simple model is the q c =2 q m lock-in term, which intertwines the magnetic and orbital modulations to form a magneto-orbital helix. Phenomenologically, different forms of the lock-in term are allowed by symmetry, with the most likely candidate involving a third-harmonic ‘squaring up’ of the magnetic modulation. Below T N1 , CaMn 7 O 12 acquires the largest measured magnetically induced electrical polarization along the c axis [4] , which can be explained by the existence of the magneto-orbital helix. CaMn 7 O 12 has point symmetry —one of the ferroaxial groups. Ferroaxiality is a ferroic property like ferroelectricity and ferromagnetism, characterized by the presence of domains having a well-defined rotation between different elements of the crystal structure. In CaMn 7 O 12 , the six oxygen atoms surrounding an individual Mn3 are all rotated in the same direction (clockwise in the domain illustrated in Fig. 4a ). The electrical polarization can arise through coupling between the chiral magneto-orbital helix and the global rotation, as described by the phenomenological invariant ασ A · P , where α is a coupling constant, σ is the magnetic helicity, P is the electrical polarization and A is an axial vector representing the structural rotation. It is important to stress that the helicity of this particular magnetic structure can be reversed by a global rotation of all the spins, so that the symmetric-exchange energy of two inversion-related domains must be the same. This implies that the spin–orbit interaction is essential to couple magnetic helicity and polarization, although striction effects can be important in achieving large values of P [17] . The relevant microscopic mechanism is the antisymmetric Dzyaloshinskii–Moriya (DM) exchange, where energy can be gained by distorting the crystal structure and/or the electronic density in the presence of non-collinear spin configurations. Although both structural and electronic distortions are allowed in the present case, we will employ the former as an illustration. When two metal sites carrying non-collinear spins are joined by common ligand atoms (in this case Mn-O-Mn), energy can be gained by displacing the ligand through a vector u so that Δ E = λ u ·[ r 12 × ( S 1 × S 2 )]= λ D ·( S 1 × S 2 ), where S 1 and S 2 are the spins on the two sites, r 12 is the position vector connecting them and λ is a coupling constant. D = u × r 12 is the familiar DM vector [18] , [19] . Energy is, therefore, minimized by a pattern of local ligand (oxygen) displacements u associated with pairs of spins and either parallel or antiparallel to the vectors r 12 × ( S 1 × S 2 ), depending on the sign of λ . 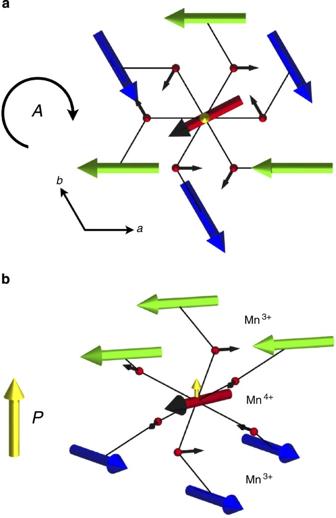Figure 4: The coupling between magnetic helicity and ferroelectricity leading to a giant polarization. (a) The global structural rotation described by the axial vectorAalong thecaxis is evident in the pattern of oxygen atoms (red spheres), which couples to the clockwise (anticlockwise) spin rotation between Mn4+and green (blue) Mn3+layers. (b) A perspective view on the Mn3+–Mn4+–Mn3+configuration. The inverse Dzyaloshinskii–Moriya interaction favours a displacement of the oxygen anions in the direction of the black arrows. This results in an additional displacement of the Mn4+cation, indicated by the small yellow arrow, and thus a net polarization along the positivecaxis, shown by the large yellow arrow. Figure 4b shows the pattern of r 12 × ( S 1 × S 2 ) vectors (black arrows) for clusters of Mn2 around a single Mn3. Assuming λ <0, the DM interaction will favour oxygen displacements parallel to these arrows, making the Mn 3+ -O-Mn 4+ bonds between the red and the blue layer flatter (that is, the bond angles closer to 180°) and Mn 3+ -O-Mn 4+ bonds between the red and the green layer more acute (that is, the bond angles farther from 180°). It is easy to see that this pattern of displacements will result in the central Mn 4+ moving upwards (yellow arrow), creating a local polarization along the positive c direction (identical considerations for λ >0 lead to a polarization along the negative c direction). As the magnetic structure is globally chiral, these local polarizations add up to give a net electrical polarization. It is important to stress that such a simple relation between local u and global P vectors is only possible in the presence of a global structural rotation, which is allowed in point-group (no net polarization would arise for 180° Mn 3+ -O-Mn 4+ bonds). Ferroaxiality is thus an essential ingredient for the development of electrical polarization in CaMn 7 O 12 . Moreover, the polarization is constrained to lie along the high-symmetry axial vector, enforcing a simple switchable 2-domain structure, where the magnetic chirality determines the direction of P (the ferroaxiality itself does not switch under applied electric field). The large value of P is readily explained by considering the angle of rotation φ between the spins S 1 and S 2 , as P should be roughly proportional to sin φ . The average angle of rotation is 〈 φ 〉=124/2°=62°, whereas for the prototypical magnetic multiferroic TbMnO 3 , φ =200°, so that sin〈 φ 〉 in CaMn 7 O 12 is 2.5 times larger than in TbMnO 3 . It is also clear to see that the small deviation from commensurability is not crucial in determining the orbital physics and the large electrical polarization in CaMn 7 O 12 : P would be almost as large if the magnetic propagation vector was exactly (0,0,1), as what matters is the large rotation angle between spins in adjacent A, B and C layers. This model should also be applicable to the complex low-temperature magnetic structure below T N2 , as the modulated structure is unaffected by the transition and the magnetic structure is still chiral. Figure 4: The coupling between magnetic helicity and ferroelectricity leading to a giant polarization. ( a ) The global structural rotation described by the axial vector A along the c axis is evident in the pattern of oxygen atoms (red spheres), which couples to the clockwise (anticlockwise) spin rotation between Mn 4+ and green (blue) Mn 3+ layers. ( b ) A perspective view on the Mn 3+ –Mn 4+ –Mn 3+ configuration. The inverse Dzyaloshinskii–Moriya interaction favours a displacement of the oxygen anions in the direction of the black arrows. This results in an additional displacement of the Mn 4+ cation, indicated by the small yellow arrow, and thus a net polarization along the positive c axis, shown by the large yellow arrow. Full size image We have shown that the magnetic and structural modulations in CaMn 7 O 12 are intertwined to form an incommensurate magneto-orbital helix. This unprecedented texture represents a novel manifestation of the deep connection between orbital physics and magnetism in transition-metal oxides. The structural modulation is crucial in stabilising a chiral magnetic structure, which breaks inversion symmetry, producing the largest magnetically induced electrical polarization ever observed in any system. We have also shown how the presence of a global structural rotation (ferroaxiality) promotes the coupling between magneto-orbital helicity and ferroelectricity. These observations open up the possibility of finding a new class of multiferroic materials in which giant ferroelectric polarizations may arise, underpinning the development of multiferroic technology. Note on magnetic propagation vector q m =(0, 0, 1.037) is equivalent to the previously reported magnetic propagation vector (0, 1, 0.963) through addition of the reciprocal lattice vector (0,1,2) to − q m . In this study, q m is chosen to lie within the first Brillouin zone of the hexagonal unit cell. Experimental details High-quality single crystals of CaMn 7 O 12 , with approximate dimensions 60 × 60 × 60 μm were grown by the flux method. A 5 g mixture of CaCl 2 :MnO 2 was heated for 25 h in an alumina crucible in air at 850 °C and then cooled at a rate of 5 °C per hour. X-ray diffraction and bulk property measurements showed that the crystals were not twinned at room temperature. Single-crystal X-ray diffraction at 150 K was performed using a SuperNova X-ray diffraction system from Agilent Technologies, fitted with an Oxford Cryosystems L N 2 cryostream. Crysalis Pro software was used for data collection and processing, enabling concurrent data reduction and identification of additional diffraction peaks that originate in the structural modulation, observed as satellites of Bragg reflections from the average structure. A powder sample was prepared by grinding single crystals, and sieving through a 35-μm mesh. This sample was used to obtain accurate lattice parameters at 150 K through X-ray powder diffraction using a Siemens D5000 diffractometer. The incommensurately modulated structure was refined using Jana (2006) software [7] with lattice parameters obtained from the X-ray powder diffraction measurement, the propagation vector obtained from single-crystal X-ray diffraction, and an initial structure taken from Sławiński et al . [3] How to cite this article: Perks, N.J., et al. Magneto-orbital helices as a route to coupling magnetism and ferroelectricity in multiferroic CaMn 7 O 12 . Nat. Commun. 3:1277 doi: 10.1038/ncomms2294 (2012).